ERG induces taxane resistance in castration-resistant prostate cancer Taxanes are the only chemotherapies used to treat patients with metastatic castration-resistant prostate cancer (CRPC). Despite the initial efficacy of taxanes in treating CRPC, all patients ultimately fail due to the development of drug resistance. In this study, we show that ERG overexpression in in vitro and in vivo models of CRPC is associated with decreased sensitivity to taxanes. ERG affects several parameters of microtubule dynamics and inhibits effective drug-target engagement of docetaxel or cabazitaxel with tubulin. Finally, analysis of a cohort of 34 men with metastatic CRPC treated with docetaxel chemotherapy reveals that ERG-overexpressing prostate cancers have twice the chance of docetaxel resistance than ERG-negative cancers. Our data suggest that ERG plays a role beyond regulating gene expression and functions outside the nucleus to cooperate with tubulin towards taxane insensitivity. Determining ERG rearrangement status may aid in patient selection for docetaxel or cabazitaxel therapy and/or influence co-targeting approaches. Taxanes are used for the treatment of patients with newly diagnosed hormone sensitive metastatic prostate cancer and for first or second line treatment of patients with metastatic castration-resistant prostate cancer (CRPC), especially for symptomatic patients, and are the only class of chemotherapy agents shown to improve survival [1] , [2] , [3] . There is significant heterogeneity in how patients respond to taxane chemotherapy and most patients with CRPC ultimately become refractory due to the development of drug resistance. The molecular basis of this heterogeneity in treatment response remains to be determined. Taxanes act by binding to the β-tubulin subunit of the α/β—tubulin heterodimer, which consists of the building block of microtubules (MTs). cytoskeletal polymers vital for a multitude of cellular functions including mitotic spindle formation, intracellular trafficking and cell signalling. One of the chief characteristics of MTs is their dynamic instability: the stochastic change from phases of subunit addition (polymerization) and subunit loss (depolymerization) [4] . Dysregulation of MT dynamics leads to a number of deleterious effects, including cellular mispolarization, aberrant motility [5] , stalled cell division [6] and even cell death [7] . Taxane binding to MTs interferes with their dynamic instability by slowing down the MT polymerization rates, stabilizing MT polymers and preventing their disassembly, which results in cell death through apoptosis [8] . Despite their widespread use, the major challenge with taxane chemotherapy is the eventual development of clinical drug resistance [9] whose underlying mechanism is poorly understood. A recent report of mass spectrometric analysis showed that the transcription factor ERG interacts with β-tubulin [10] , but the biological relevance of this interaction remains uncharacterized. ERG is overexpressed by 30- to 80-fold in at least 50% of prostate cancers as a result of recurrent gene fusions, driven by one of three 5′ promoters (that is, TMPRSS2 , SLC45A3 and NDRG1 ) [11] . ERG rearrangement represents an early event in prostate cancer tumorigenesis [12] , and, although other somatic alterations have been described in critical pathways (for example, PI3K/PTEN, RB and RAS/RAF [13] ), ERG rearrangement represents the most frequent recurrent genetic alteration in prostate cancer. In vivo and in vitro data support a causal role of ERG in initiating prostate epithelial transformation (in cooperation with other molecular alterations) and in increasing cell invasion [14] , [15] . Recent data have shown that ERG contributes genome-wide by reorganizing the chromatin within the nucleus and facilitating both the formation of pro-malignancy transcription hubs and influencing the development of other genomic alterations [16] , [17] . Herein, we show that ERG overexpression is associated with decreased taxane sensitivity in prostate cancer cell lines, in vivo xenograft models, and in ERG-positive CRPC patients. Mechanistically, we show that ERG contributes to taxane resistance by binding soluble tubulin in the cytoplasm, altering microtubule dynamics towards increased catastrophe rate, and thereby shifting the dynamic equilibrium between microtubule polymers (preferred taxane substrate) and soluble tubulin dimers (preferred substrate for MT-depolymerizing drugs) towards soluble tubulin. This shift, in turn, renders cells resistant to taxanes but more sensitive to microtubule depolymerizing drugs. Taken together, our data support a novel cytoplasmic function of ERG and suggest that ERG may be a potential predictive biomarker of taxane response in prostate cancer patients. ERG overexpression leads to taxane-resistance in vitro To test whether ERG expression has an impact on taxane sensitivity, we used siRNA (siERG) to lower ERG levels in the VCaP cells, which endogenously express the TMPRSS2-ERG fusion [11] , and measured cell viability following 72 h of cabazitaxel treatment. Reduced ERG levels resulted in an increase in cabazitaxel sensitivity compared with control cells transfected with a scrambled siRNA molecule (siSCR, Fig. 1a ). To extend these observations, we generated isogenic cell lines with stable [14] , [17] or inducible ERG expression. Stable ERG overexpression reproducibly resulted in a markedly lower sensitivity to cabazitaxel in RWPE1 ( Supplementary Fig. 1a ) and DU145 independent cell clones while knocking down ERG in the DU145 cells with stable ERG overexpression (DU145-ERG) using an shRNA restored their sensitivity ( Fig. 1b ). Increasing levels of ERG using tetracycline (TetOn)-inducible DU145 cells led to a dose-dependent decrease in cabazitaxel sensitivity compared with the same cell line in the absence of doxycycline or doxycycline-treated TetOn-empty vector control cells ( Fig. 1c , Supplementary Fig. 1b ). In addition, ERG overexpression in DU145 cells conferred resistance to cabazitaxel-induced apoptosis, measured by caspase 3/7 activity in a time- and dose-dependent manner ( Fig. 1d–f ). Induced ERG overexpression also conferred docetaxel resistance ( Supplementary Fig. 1c,d ). Taken together these data show that ERG overexpression leads to taxane (cabazitaxel and docetaxel) resistance in vitro , proportional to the amount of ERG expression, and that ERG knockdown sensitizes cells to taxane treatment. 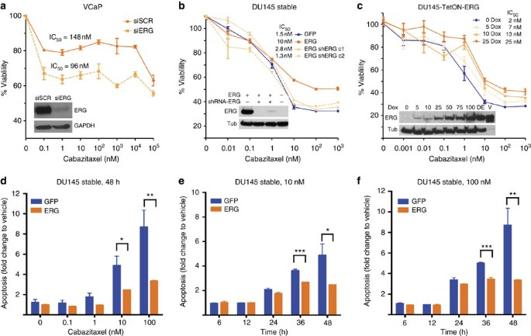Figure 1: ERG overexpression leads to taxane resistancein vitro. (a) Dose–response curves following a 72-h incubation at the indicated dose of cabazitaxel for VCaP cells with ERG knockdown (siERG) or scramble knockdown (siSCR), as a control. Inset: immunoblot showing ERG protein expression with GAPDH as a loading control. Dose–response curves following a 48 h incubation at the indicated dose of cabazitaxel for DU145 clones stably overexpressing ERG (orange) or GFP (blue) (b) or with doxycycline (dox)-inducible ERG expression (TetON-ERG) (c). Insets: immunoblot showing ERG protein expression with tubulin as a loading control. (d–f) Apoptosis induction (caspase 3/7 activity) at 48 h as a function of cabazitaxel dose (d) or at the indicated time points (hours) in the presence of either 10 nM (e) or 100 nM cabazitaxel (f) of DU145 cells stably expressing GFP (blue) or ERG (orange). Values are normalized to vehicle-treated cells at the indicated time point. *(Pvalue <0.01), **(Pvalue <0.005) or ***(Pvalue <0.0002) based onT-tests. Western blot images have been cropped for presentation. Full-size images are presented inSupplementary Fig. 11. Figure 1: ERG overexpression leads to taxane resistance in vitro. ( a ) Dose–response curves following a 72-h incubation at the indicated dose of cabazitaxel for VCaP cells with ERG knockdown (siERG) or scramble knockdown (siSCR), as a control. Inset: immunoblot showing ERG protein expression with GAPDH as a loading control. Dose–response curves following a 48 h incubation at the indicated dose of cabazitaxel for DU145 clones stably overexpressing ERG (orange) or GFP (blue) ( b ) or with doxycycline (dox)-inducible ERG expression (TetON-ERG) ( c ). Insets: immunoblot showing ERG protein expression with tubulin as a loading control. ( d – f ) Apoptosis induction (caspase 3/7 activity) at 48 h as a function of cabazitaxel dose ( d ) or at the indicated time points (hours) in the presence of either 10 nM ( e ) or 100 nM cabazitaxel ( f ) of DU145 cells stably expressing GFP (blue) or ERG (orange). Values are normalized to vehicle-treated cells at the indicated time point. *( P value <0.01), **( P value <0.005) or ***( P value <0.0002) based on T -tests. Western blot images have been cropped for presentation. Full-size images are presented in Supplementary Fig. 11 . Full size image ERG overexpression leads to taxane resistance in vivo To determine whether ERG lowers the sensitivity of tumour cells to taxanes in vivo , different clonal populations of luciferase-expressing DU145-ERG cells or control DU145 cells expressing the empty vector (DU145-GFP) were used to generate xenografts as previously described [18] . Tumours were allowed to grow to an average tumour volume of 150 mm 3 . For each study, five tumour-bearing mice were randomized to treatment (intraperitoneal dosing of 12 mg kg −1 cabazitaxel every 6 days for 4 weeks) or vehicle groups. DU145-ERG xenografts were reproducibly more resistant to cabazitaxel compared with the cabazitaxel-sensitive control xenografts based on both tumour volume as measured using a caliper and tumour cell viability as measured using bioluminescent imaging ( Fig. 2 and Supplementary Fig. 2a,b ). ERG overexpression did not affect tumour growth rate appreciably compared with control tumours ( Supplementary Fig. 2c ). Body weight decreased on average by 8% at week 5 in mice with control tumours, which was somewhat abrogated in mice with ERG expressing tumours with a 3% average ( Supplementary Fig. 2d ). In summary, these results show that ERG overexpression leads to taxane resistance in vivo, similar to what was observed in vitro . 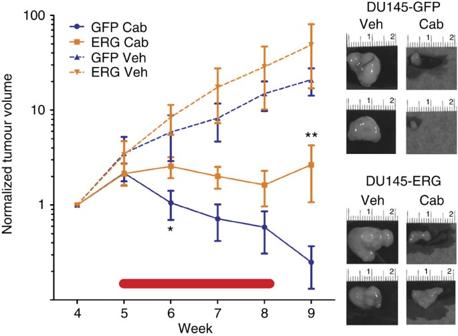Figure 2: ERG overexpression leads to taxane resistancein vivo. DU145-ERG (orange) or DU145-GFP (blue) tumour xenograft volume assessment (average±s.e.m.) before, during (red line) and after treatment with 48 mg kg−1cabazitaxel (Cab, solid lines) or vehicle (Veh, dashed lines) at the indicated week following cell subcutaneous injection (n=5 mice/group). All values were normalized to the average tumour size per group at the time that the mice were randomized into the indicated groups. Images are representative of tumours at week 10 from each of the four groups (+/− ERG and treated with cabazitaxel or vehicle). *(Pvalue=0.07) and ***(Pvalue=0.006) based onT-tests comparing DU145-ERG cabazitaxel-treated group with DU145-GFP cabazitaxel treated. Figure 2: ERG overexpression leads to taxane resistance in vivo . DU145-ERG (orange) or DU145-GFP (blue) tumour xenograft volume assessment (average±s.e.m.) before, during (red line) and after treatment with 48 mg kg −1 cabazitaxel (Cab, solid lines) or vehicle (Veh, dashed lines) at the indicated week following cell subcutaneous injection ( n =5 mice/group). All values were normalized to the average tumour size per group at the time that the mice were randomized into the indicated groups. Images are representative of tumours at week 10 from each of the four groups (+/− ERG and treated with cabazitaxel or vehicle). *( P value=0.07) and ***( P value=0.006) based on T -tests comparing DU145-ERG cabazitaxel-treated group with DU145-GFP cabazitaxel treated. Full size image ERG impairs effective drug-target engagement of MTs Taxanes bind to and stabilize interphase and mitotic spindle MTs impairing their normal function and inducing apoptosis [19] . To investigate whether ERG overexpression had any effect on the ability of cabazitaxel to engage its target, we examined the extent of drug-induced microtubule stabilization in the isogenic ERG-negative and-positive DU145 cells using a cell-based tubulin polymerization assay. This assay provides a quantitative output for the dynamic equilibrium between the pool of soluble tubulin dimers (S) and microtubule polymers (P) in untreated cells as well as any drug-induced shifts of this equilibrium in cells treated with MT inhibitors [20] , [21] , [22] . Cells were treated with cabazitaxel at either the IC 50 concentration (1 nM)—a physiologically relevant drug concentration corresponding to the steady-state serum levels of cabazitaxel achieved clinically in CRPC patients- or the supra- physiological 10 × IC 50 (10 nM) concentration. Treatment of the DU145-ERG negative cells resulted in a dose-dependent induction of tubulin polymerization from 17% polymer (P) in the control untreated cells to 31% P and 81% P following treatment with 1 and 10 nM cabazitaxel, respectively ( Fig. 3a ). In contrast, treatment of DU145-ERG-positive cells with the IC 50 concentration of cabazitaxel had no effect of tubulin polymerization (10% P in control versus 8% P at 1 nM), indicating impaired drug-target engagement (DTE). As expected, this impairment was abrogated following treatment with the supra-physiological 10 nM dose of cabazitaxel. 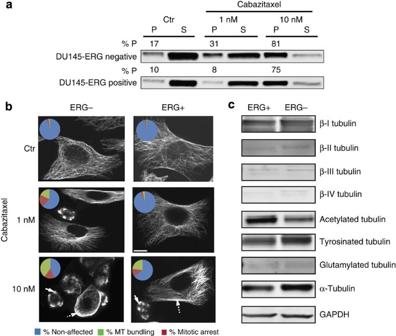Figure 3: Assessment of effective drug-target engagement. DU145 ERG-negative or ERG-positive cells were treated with the indicated drug concentrations for 24 h and processed for tubulin polymerization assay (a) or indirect immunofluorescence followed by confocal microscopy (b). (a) Following cabazitaxel treatment, cells were lysed with a hypotonic buffer, and the polymerized (P) and soluble (S) tubulin fractions were separated by centrifugation. Equal volumes from each fraction were loaded on adjacent wells of an SDS/PAGE and immunoblotted with an antibody against α-tubulin. The percent of polymerized tubulin (%P) was determined by dividing the densitometric value of polymerized tubulin by the total tubulin content (the sum of P plus S). (b) Following cabazitaxel treatment, cells were fixed and processed for tubulin immunofluorescent staining and imaged by confocal microscopy. Cells were then assessed for the presence of effective drug-induced microtubule stabilization, as in microtubule bundling (dashed arrows) or aberrant mitotic arrest (solid arrows). Representative cells are shown from each condition. Pie chart inset shows graphically the percent of cells that showed no drug effect (blue), MT bundling (green) or mitotic arrest (red). Scale bar, 10 μm. Cell counts andP-values calculated from Fischer exact tests are shown graphically below for each condition. Cells arrested in mitosis or with visible MT bundling are considered cabazitaxel affected and thus grouped together (orange bars), unaffected cells are depicted in blue bars. (c) Expression profile of different β-tubulin isotypes and post-translational modifications in ERG-positive and ERG-negative cells. Equal amounts of protein from each condition (50 μg) were loaded on SDS–PAGE and separated through electrophoresis; GAPDH was used as a loading control. Representative images of biological triplicated are shown. Western blot images have been cropped for presentation. Full-size images are presented inSupplementary Fig. 11. Figure 3: Assessment of effective drug-target engagement. DU145 ERG-negative or ERG-positive cells were treated with the indicated drug concentrations for 24 h and processed for tubulin polymerization assay ( a ) or indirect immunofluorescence followed by confocal microscopy ( b ). ( a ) Following cabazitaxel treatment, cells were lysed with a hypotonic buffer, and the polymerized (P) and soluble (S) tubulin fractions were separated by centrifugation. Equal volumes from each fraction were loaded on adjacent wells of an SDS/PAGE and immunoblotted with an antibody against α-tubulin. The percent of polymerized tubulin (%P) was determined by dividing the densitometric value of polymerized tubulin by the total tubulin content (the sum of P plus S). ( b ) Following cabazitaxel treatment, cells were fixed and processed for tubulin immunofluorescent staining and imaged by confocal microscopy. Cells were then assessed for the presence of effective drug-induced microtubule stabilization, as in microtubule bundling (dashed arrows) or aberrant mitotic arrest (solid arrows). Representative cells are shown from each condition. Pie chart inset shows graphically the percent of cells that showed no drug effect (blue), MT bundling (green) or mitotic arrest (red). Scale bar, 10 μm. Cell counts and P -values calculated from Fischer exact tests are shown graphically below for each condition. Cells arrested in mitosis or with visible MT bundling are considered cabazitaxel affected and thus grouped together (orange bars), unaffected cells are depicted in blue bars. ( c ) Expression profile of different β-tubulin isotypes and post-translational modifications in ERG-positive and ERG-negative cells. Equal amounts of protein from each condition (50 μg) were loaded on SDS–PAGE and separated through electrophoresis; GAPDH was used as a loading control. Representative images of biological triplicated are shown. Western blot images have been cropped for presentation. Full-size images are presented in Supplementary Fig. 11 . Full size image This impaired DTE was further confirmed by confocal microscopy using two additional readouts, MT bundling and abnormal multipolar spindle formation, both of which represent hallmarks of cellular taxane activity. The ability of cabazitaxel to induce microtubule bundling ( Fig. 3b , dashed arrows) and/or aberrant mitotic arrest ( Fig. 3b , solid arrows) was significantly compromised in ERG-positive cells, as compared with the extent of DTE observed in ERG-negative cells ( Fig. 3b and Supplementary Fig. 3a ). Furthermore, we did not detect any ERG-specific significant differences in β-tubulin isotype expression or post-translational modifications associated with microtubule stability, such as acetylation, tyrosination and glutamylation [23] , [24] , [25] , between ERG-negative and ERG-positive cells ( Fig. 3c and Supplementary Fig. 3b ). Finally, to ensure that there was no reduction in the intracellular accumulation of cabazitaxel in ERG+ cells due to overexpression of the cell surface efflux pump P-glycoprotein (P-gp) [26] , [27] , [28] , we quantitatively assessed P-gp protein expression by flow cytometry. No P-gp was detected in ERG+ or ERG− cells, indicating that this mechanism is not involved in the observed taxane resistance phenotype ( Supplementary Fig. 4a ). In addition, to rule out other potential mechanisms of active drug transport, we performed drug accumulation assays using radiolabelled 14 C-cabazitaxel and found no difference in the intracellular drug accumulation between the ERG+ and ERG− cells ( Supplementary Fig. 4b ). Taken together, these results indicate that ERG overexpression in prostate cancer cells renders MTs less responsive to taxane treatment suggesting that the drug–tubulin interaction might be compromised under these conditions. Dynamic MTs are critical for cell division, intracellular transport and cell signalling, and it has been shown that taxane treatment causes significant perturbation of microtubule dynamics in vitro and in vivo [19] . To test whether ERG expression interferes with microtubule dynamics in prostate cancer cells, we measured MT dynamics in living cells fluorescently tagged EB1 (end-binding protein 1), a protein that binds only to the growing tip of the polymerizing MT and is used as a marker for the direct visualization of MT polymerization dynamics [29] , [30] . We obtained time-lapse images of untreated or docetaxel-treated cells using high-resolution confocal microscopy ( Supplementary Videos 1–4 ) and performed computational analysis of MT dynamics using an automated motion-tracking algorithm [31] . We analysed over 10,000 MT growth tracks across multiple cells from each condition and obtained quantitative readouts of 12 different parameters of MT dynamics ( Supplementary Tables 1 and 2 ). This analysis revealed that MTs in ERG expressing cells are less responsive to the stabilizing effects of docetaxel as compared with MTs in ERG-negative cells across multiple parameters of MT dynamics (for example, growth track, gap/pause, shrinkage and growth segment speeds ( Fig. 4 , Supplementary Fig. 5 and Supplementary Table 1 ). Importantly, ERG overexpression significantly reduced three parameters of MT dynamics in untreated cells ( Supplementary Table 1 ), all of which signify increased catastrophe frequency in ERG-positive cells. Together, these results show that ERG expression affects microtubule homeostasis and dynamics at baseline influencing their responsiveness to taxane treatment. 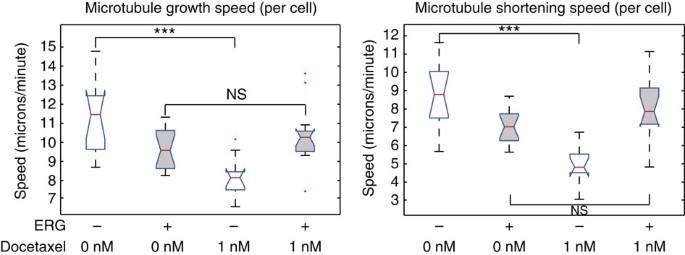Figure 4: ERG impacts microtubule dynamics. Analysis of MT dynamics using EB1-EGFP live cell imaging and computational tracking of individual EB1 comets. Bar charts of directly measured growth speeds (left) or computationally inferred shortening speeds of >2,000 MTs imaged across multiple DU145-ERG or DU145-GFP cells, either untreated (ctr) or treated with 1 nM docetaxel. Figure 4: ERG impacts microtubule dynamics. Analysis of MT dynamics using EB1-EGFP live cell imaging and computational tracking of individual EB1 comets. Bar charts of directly measured growth speeds (left) or computationally inferred shortening speeds of >2,000 MTs imaged across multiple DU145-ERG or DU145-GFP cells, either untreated (ctr) or treated with 1 nM docetaxel. Full size image ERG directly interacts with tubulin Although ERG is primarily a nuclear protein [32] , it has also been detected in the cytoplasm in a subset of prostate cancer cells ( Supplementary Fig. 6a ). In addition, a recent report of mass spectrometric analysis of ERG-interacting proteins showed that ERG interacts with β-tubulin [10] . Thus, to investigate whether ERG affected MT dynamics, indirectly by altering gene transcription or more directly by physically interacting with tubulin in the cytoplasm, we performed co-immunoprecipitation (co-IP) and MT co-sedimentation assays in ERG+ and ERG– cells. We found that tubulin was specifically co-precipitated with ERG in VCaP (endogenous ERG) or DU145-ERG (exogenous ERG) cells ( Fig. 5 ). The specificity of this interaction was confirmed following reverse co-IP using an antibody against α-tubulin (DM1a). These data suggest that ERG-induced taxane resistance and altered MT dynamics may be resultant, in part, of a direct interaction between ERG and tubulin. To identify the ERG domain mediating the tubulin association, we performed ERG/tubulin co-IP in DU145-GFP cells transiently transfected with flag-tagged ERG expression vectors encoding either wild-type TMPRSS2-ERG (encoding truncated ERG) or tiling deletion mutants [10] that are devoid of key functional domains (for example, pointed (PNT), CAE/CD, transactivating or ETS DNA binding [33] , [34] , Fig. 5b ). These exogenously introduced ERG variants were lacking the following domains: N terminus (aa 47–115, predicted molecular weight 44.6 kDa, ΔN); PNT domain (aa 115–197, 43.4 kDa, ΔP); the middle amino acids that correspond to the CAE/CD domain (197–310, 41.6 kDa, ΔM); the ETS (aa 310–393, 43.7 kDa, ΔE) or the transactivating C terminus (aa 393–479, 43.6 kDa, ΔC) ( Fig. 5b ). Using the Flag antibody to precipitate each of the variants, we found that tubulin was co-immunoprecipitated with all of the ERG mutant variants except the one lacking the PNT domain (ΔP), suggesting that this domain is essential for the ERG–tubulin interaction ( Fig. 5c ). We found no interaction between wild-type ERG or any of the ERG variants and other abundant structural and non-structural cytoplasmic proteins (for example, keratins, GAPDH, Supplementary Fig. 6c ). Importantly, the lack of the ERG–tubulin interaction in ΔP expressing cells restored sensitivity to taxanes ( Fig. 5e ). 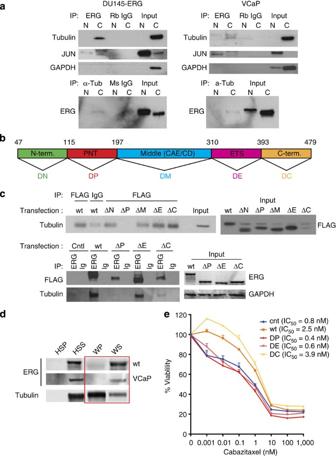Figure 5: ERG interacts with tubulin. (a) Co-immunoprecipitation (IP) of purified cytoplasmic or nuclear cell fractions using an anti-ERG or anti α-tubulin antibody followed by immunoblot for the indicated proteins in DU145-ERG cells or in VCaP cells. For all experiments isotype-matched IgGs were used to control for non-specific binding to the beads used for immunoprecipitation. (b) Graphic representation of the full-length TMPRSS2-ERG encoded protein with the different domains colour coded as follows (green, N terminus (ΔN); red, pointed domain (ΔP); blue, the middle amino acids that correspond to the CAE/CD domain (ΔM); pink, the ETS domain (ΔE); gold, C terminal transactivating domain (ΔC)). (c) Co-immunoprecipitation (IP) of whole-cell extracts from DU145-GFP, 72 h following transient transfection with the Flag-tagged wild type or indicated deletion ERG constructs using either anti-Flag or anti-ERG antibody followed by immunoblot for the indicated proteins. Isotype-matched IgGs were used to control for non-specific binding to the beads used for immunoprecipitation. Immunoblot of input lysate for each transfection are shown to the left of each IP blot. (d) Microtubule co-sedimentation assay of DU145 cells transiently expressing ERG-WT (wt) or Vcap cells expressing endogenous ERG protein. One mg of precleared cell lysate from each condition (HSS) was supplemented with exogenous purified tubulin and subjected to a cycle of polymerization in presence of GTP and paclitaxel at 37 °C. The samples were centrifuged at 100,000 ×gto separate the microtubule polymers (WP) from the soluble tubulin dimers (WS), resolved by SDS–PAGE and immunoblotted for ERG and tubulin. HSP=high-speed pellet (containing cellular debris and nonspecific protein aggregates); HSS=high-speed supernatant (precleared cell lysate); WP=warm pellet containing microtubule polymers; WS=warm supernatant containing soluble tubulin dimers. (e) Cell viability assay of the indicated DU145 cells transiently expressing each of the ERG deletion mutants as in (c) in response to 48 h treatment with cabazitaxel. Western blot images have been cropped for presentation. Full-size images are presented inSupplementary Fig. 12. Figure 5: ERG interacts with tubulin. ( a ) Co-immunoprecipitation (IP) of purified cytoplasmic or nuclear cell fractions using an anti-ERG or anti α-tubulin antibody followed by immunoblot for the indicated proteins in DU145-ERG cells or in VCaP cells. For all experiments isotype-matched IgGs were used to control for non-specific binding to the beads used for immunoprecipitation. ( b ) Graphic representation of the full-length TMPRSS2-ERG encoded protein with the different domains colour coded as follows (green, N terminus (ΔN); red, pointed domain (ΔP); blue, the middle amino acids that correspond to the CAE/CD domain (ΔM); pink, the ETS domain (ΔE); gold, C terminal transactivating domain (ΔC)). ( c ) Co-immunoprecipitation (IP) of whole-cell extracts from DU145-GFP, 72 h following transient transfection with the Flag-tagged wild type or indicated deletion ERG constructs using either anti-Flag or anti-ERG antibody followed by immunoblot for the indicated proteins. Isotype-matched IgGs were used to control for non-specific binding to the beads used for immunoprecipitation. Immunoblot of input lysate for each transfection are shown to the left of each IP blot. ( d ) Microtubule co-sedimentation assay of DU145 cells transiently expressing ERG-WT (wt) or Vcap cells expressing endogenous ERG protein. One mg of precleared cell lysate from each condition (HSS) was supplemented with exogenous purified tubulin and subjected to a cycle of polymerization in presence of GTP and paclitaxel at 37 °C. The samples were centrifuged at 100,000 × g to separate the microtubule polymers (WP) from the soluble tubulin dimers (WS), resolved by SDS–PAGE and immunoblotted for ERG and tubulin. HSP=high-speed pellet (containing cellular debris and nonspecific protein aggregates); HSS=high-speed supernatant (precleared cell lysate); WP=warm pellet containing microtubule polymers; WS=warm supernatant containing soluble tubulin dimers. ( e ) Cell viability assay of the indicated DU145 cells transiently expressing each of the ERG deletion mutants as in ( c ) in response to 48 h treatment with cabazitaxel. Western blot images have been cropped for presentation. Full-size images are presented in Supplementary Fig. 12 . Full size image ERG interacts with soluble tubulin dimers Several proteins interact with tubulin either in its soluble form of αβ-heterodimers (for example, stathmin [35] ) or in its polymerized form of microtubule filaments (for example, androgen receptor, p53) [36] , [37] . To evaluate whether ERG interacts with soluble tubulin or MTs, we performed a microtubule co-sedimentation assay, in which cell lysates are incubated with purified tubulin, GTP and paclitaxel and are subjected to a cycle of polymerization at 37 °C. Following ultracentrifugation, the MT polymers and all cellular proteins with affinity for them sediment together in the same fraction as the polymerized tubulin (WP), while the soluble pool of tubulin dimers remains in the supernatant (WS). Figure 5d shows the results of the MT co-sedimentation assay performed using either cells expressing endogenous ERG (VCaP) or DU145 cells transiently transfected with exogenous wild-type ERG. Immunoblot analysis revealed that, although the majority of tubulin was found in the polymer fraction as expected under the assay conditions, ERG protein was detected predominantly in the supernatant (WS fraction), indicating that ERG predominantly interacts with tubulin dimers as opposed to MT polymers ( Fig. 5d ). ERG impairs taxane binding ability to MTs To evaluate whether ERG overexpression interferes with taxane binding to MTs, we treated live ERG-positive and ERG-negative DU-145 cells with fluorescently labelled paclitaxel (Flutax) and monitored the extent and stability of Flutax binding to the microtubule network [38] . We found that the ERG-positive DU145 cells had significantly fewer MTs labelled with Flutax as compared with ERG-negative cells, in which Flutax labelled an extensive and intricate microtubule network throughout the cell cytoplasm ( Supplementary Fig. 7a,b ). Importantly, in ERG-positive cells, Flutax labelled only a few short MTs emanating from the centrosome, site of microtubule nucleation, while there was very sparse if any microtubule labelling towards the cell periphery ( Supplementary Fig. 7c (see yellow trace of cellular outline)). Furthermore, the ability of Flutax to change its fluorescent intensity and anisotropy as a result of microtubule binding makes it an outstanding tool to monitor binding affinity and has been extensively used in microtubule binding kinetics and affinity studies [39] . Thus, to test whether ERG overexpression had any effect on the kinetics of Flutax binding to cellular MTs, we monitored the dissociation kinetics of Flutax in a time course drug-wash out experiment. Our results showed that Flutax’s labelling of MTs in ERG-positive cells was both significantly lower across time points ( Fig. 6a,c ), as well as less durable in comparison with ERG-negative cells ( Fig. 6b ). Together these results indicate impaired and transient binding of Flutax to MTs in the presence of ERG overexpression. 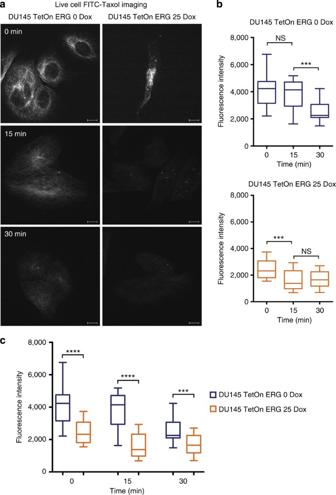Figure 6: ERG impairs taxane binding ability to microtubules. (a) Live cell FITC-Taxol immunofluorescence. Live ERG-positive and ERG-negative DU145 cells were permeabilized with 0.5% Triton X-100 and treated with 1 μM FITC-labelled paclitaxel for 5 min. Images of live cells were subsequently acquired with confocal microscope ( × 63/1.4NA objective, Zeiss, Germany) after 0, 15 and 30 min from the treatment. Representative images are shown for each condition. Scale bar, 10 μM. (b,c) Graphic representation of quantification of fluorescence intensity from (a); quantification of fluorescence intensity of an average of 30 cells per condition was done using MetaMorph image analysis software (Molecular Device, CA, USA). Figure 6: ERG impairs taxane binding ability to microtubules. ( a ) Live cell FITC-Taxol immunofluorescence. Live ERG-positive and ERG-negative DU145 cells were permeabilized with 0.5% Triton X-100 and treated with 1 μM FITC-labelled paclitaxel for 5 min. Images of live cells were subsequently acquired with confocal microscope ( × 63/1.4NA objective, Zeiss, Germany) after 0, 15 and 30 min from the treatment. Representative images are shown for each condition. Scale bar, 10 μM. ( b , c ) Graphic representation of quantification of fluorescence intensity from ( a ); quantification of fluorescence intensity of an average of 30 cells per condition was done using MetaMorph image analysis software (Molecular Device, CA, USA). Full size image ERG is associated with taxane resistance in CRPC patients To test whether clinical ERG overexpression affects the response of prostate cancer patients to standard of care taxane chemotherapy, we assessed the expression of the TMPRSS2-ERG translocation by FISH and ERG protein by IHC in a cohort of men with metastatic castrate-resistant prostate cancer treated with docetaxel chemotherapy. A strong association (95.7% sensitivity and 96.5% specificity) between ERG gene rearrangement and truncated ERG protein product expression has previously been shown [32] . While ERG status was assessed in the primary tumour, it has been shown that ERG is expressed at comparable levels in ERG-rearranged hormone-naive prostate cancer and CRPC [14] , [40] including the initial index case [11] and in circulating tumour cells (CTCs) [41] . Moreover, a recent study found a 97% concordance of ETS status between primary prostate cancer and matched metastatic site [42] . Of the 34 cases, 11 were TMPRSS2 ERG-positive ( Table 1 , Supplementary Fig. 8a ). In the overall cohort, 23/28 (68%) showed PSA response according to PCWG2 criteria ( Table 1 and Supplementary Table 3 ). Of the patients who were TMPRSS2 ERG-positive, 45% showed PSA response to docetaxel therapy compared with 79% in TMPRSS2 ERG-negative patients ( P =0.056, odds ratio=0.23 (0.05–1.09 95% confidence interval), X 2 -test) ( Table 1 and Supplementary Table 3 ), which can be appreciated in the waterfall plot of the greatest percent change in serum PSA during docetaxel treatment ( Supplementary Fig. 8b ). Although these differences did not quite reach statistical significance due to the small numbers, they suggest that docetaxel resistance is twice as likely in TMPRSS2 ERG-positive CRPC than in TMPRSS2 ERG-negative prostate cancers. Table 1 The proportion of metastatic CRPC patients showing maximal PCWG2 PSA response to docetaxel. Full size table ERG impairs taxane engagement in CTCs To further evaluate the potential role of ERG in diminishing taxane engagement in clinical samples, we isolated CTCs from patients with metastatic CRPC using the geometrically enhanced differential immunocapture (GEDI) microfluidic device [43] . Viable CTCs captured using this GEDI device can be treated ex vivo with taxanes to assess effective DTE based on the presence of microtubule bundling as hallmark of taxane on-target stabilizing activity. The presence of bundling strongly correlates with patient clinical response to taxane-based chemotherapy [43] . Here, we isolated viable CTCs from two CRPC patients whose primary tumours had confirmed positive or negative ERG rearrangement status. The isolated CTCs were treated ex vivo with each of the two clinically used taxanes, docetaxel or cabazitaxel, and processed for DTE assessment following multiplex confocal microscopy ( Supplementary Fig. 9 ). In CTCs captured from the ERG-negative patient, we observed robust DTE in 41 of the 66 captured CTCs (62%) and in 82 of the 105 captured CTCs (78%) following docetaxel and cabazitaxel treatment, respectively. In contrast, in the CTCs isolated from the ERG-positive patient, there was no increase in microtubule bundling with either treatment. Although antibody-based CTC approaches are limited in that they enrich for only those cells that express the antigen of choice [44] , these results show that CTCs isolated from mCRPC patients show differential taxane response according to ERG expression. In summary, these results extend our clinical observations in the retrospective clinical analyses ( Table 1 and Supplementary Table 3 ) and support a new role of ERG protein expression as a biomarker predictive of clinical resistance to taxane-based chemotherapy in CRPC patients, especially given that ERG expression is maintained in following ADT [14] , [40] . Work from multiple independent investigations have shown that ERG plays a driving role in cell invasion [14] , [15] , [45] , [46] , [47] , prostate tumorigenesis [15] , [45] , [46] , [48] , [49] , [50] , altered AR signalling [48] , [51] , DNA repair [10] , chromatin topology [17] and is associated with a specific translocation pattern [52] , [53] . Here we show, for the first time, that ERG overexpression is directly associated with decreased sensitivity to taxane chemotherapy in vitro and in vivo providing new data related to molecular changes that may underlie the clinical variability seen among prostate cancer patients’ response to taxane chemotherapy. These data are particularly timely based on recent findings from the NIH-supported randomized controlled clinical trial (E3805, CHAARTED: ChemoHormonal Therapy Versus Androgen Ablation Randomized Trial for Extensive Disease in Prostate Cancer) [54] . This study demonstrated that men with hormone-sensitive metastatic prostate cancer who received docetaxel chemotherapy given at the time of standard androgen deprivation (ADT) therapy lived more than a year longer than patients who received hormone therapy alone. This median difference in overall survival of greater than a year is significantly longer than any previous randomized phase III trial with any therapy and further validates the benefit of docetaxel in advanced prostate cancer. Taxanes inhibit MT dynamics and alter the spatial organization of the MT network, thereby inhibiting intracellular trafficking and signalling pathways critical for tumour survival. We found that ERG affects microtubule dynamics, binds to the soluble pool of αβ-tubulin dimers and shifts the MT polymer, dimer equilibrium towards the soluble pool of tubulin dimers ( Fig. 7 ). As the MT polymer is the preferred substrate for taxane binding, ERG expression confers drug resistance by reducing the presence of available substrate binding sites. Similarly, the ERG-induced increase in tubulin dimers renders cells sensitive to the effects of microtubule depolymerizing drugs, known to bind preferentially to the tubulin dimer ( Fig. 7 ). Indeed, treatment with the depolymerizing drugs nocodazole or Eribulin [55] revealed lack of resistance or even enhanced sensitivity in ERG-positive cells as compared with their ERG-negative counterparts ( Supplementary Fig. 10 ). Treatment with the DNA-damaging drug cisplatin did not show any significant difference in drug sensitivity as a function of ERG status, while increasing levels of ERG protein expression using the tetracycline (TetOn)-inducible DU145 cells led to a dose-dependent increase in nocodazole sensitivity ( Supplementary Fig. 10c ) which is the exact opposite result compared with that obtained with cabazitaxel treatment. Taken together these data support a new role for ERG as a microtubule-destabilizing MAP, similar to stathmin [35] , but with important therapeutic implications for prostate cancer treatment. Similar to our own findings with ERG expression, stathmin increases the catastrophe rate of MTs by binding to tubulin heterodimers sequestering them away from the MT, thereby acting as a prominent MT destabilizer. In addition, stathmin overexpression has been clearly associated with increased local invasion and metastasis formation, increased cell motility and cancer progression across many different tumour types [56] . Importantly, several studies have shown that stathmin expression mediates taxane resistance, while conferring sensitivity to vinca alkaloids as stathmin binding to tubulin dimers increases significantly the vinblastine binding affinity for tubulin [57] . Similarly, mutations identified in the MT-associated protein TEKT4 in a cohort of breast cancer patients were shown reduced MT stability and were associated with shorter disease-free survival and overall survival in patients undergoing taxane-based chemotherapy [58] . 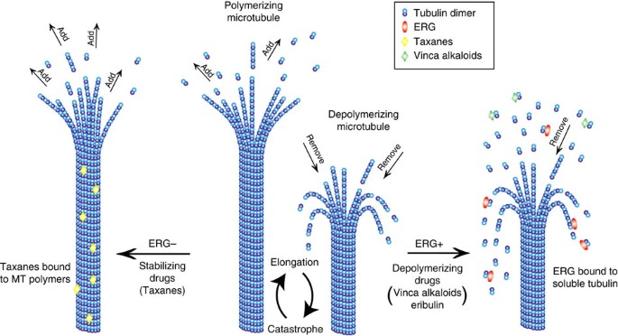Figure 7: Working model of ERG-mediated taxane resistance in prostate cancer. Microtubules are cytoskeletal filaments made of the head-to-tail association of αβ tubulin heterodimers. Microtubules exist in cells in a dynamic equilibrium between their polymerized form (MTs) and soluble form of tubulin dimers. Microtubules undergo cycles of elongation (during which new αβ tubulin dimers are added to the growing protofilaments resulting in an elongation of the microtubule polymer) and catastrophe (during which the tubulin dimers are released from the polymer, resulting in the shortening of the microtubule). In ERG-negative PC cells, microtubule stabilizing drugs (that is, taxanes) bind to the microtubule polymer, which is their preferred substrate and stabilize MTs by promoting their elongation and by preventing the removal of tubulin dimers (depolymerization). In ERG- positive PC cells, ERG binds tubulin dimers, and sequesters them away from the MT polymers, promoting microtubule catastrophe and increasing the pool of soluble tubulin dimers, which are the preferred substrate of microtubule depolymerizing drugs (that is, Vinca Alkaloids, Eribulin). Thus, ERG expression confers resistance to taxane chemotherapy, but sensitivity to microtubule destabilizing drugs. Figure 7: Working model of ERG-mediated taxane resistance in prostate cancer. Microtubules are cytoskeletal filaments made of the head-to-tail association of αβ tubulin heterodimers. Microtubules exist in cells in a dynamic equilibrium between their polymerized form (MTs) and soluble form of tubulin dimers. Microtubules undergo cycles of elongation (during which new αβ tubulin dimers are added to the growing protofilaments resulting in an elongation of the microtubule polymer) and catastrophe (during which the tubulin dimers are released from the polymer, resulting in the shortening of the microtubule). In ERG-negative PC cells, microtubule stabilizing drugs (that is, taxanes) bind to the microtubule polymer, which is their preferred substrate and stabilize MTs by promoting their elongation and by preventing the removal of tubulin dimers (depolymerization). In ERG- positive PC cells, ERG binds tubulin dimers, and sequesters them away from the MT polymers, promoting microtubule catastrophe and increasing the pool of soluble tubulin dimers, which are the preferred substrate of microtubule depolymerizing drugs (that is, Vinca Alkaloids, Eribulin). Thus, ERG expression confers resistance to taxane chemotherapy, but sensitivity to microtubule destabilizing drugs. Full size image Our findings on ERG together with the published literature on the effects of various MAPs affecting MT homeostasis and stability highlight the need to better understand cellular factors and pathways affecting MT integrity, dynamics and function to rationally customize chemotherapy to the individual. Our working model ( Fig. 7 ) suggests that patients with ERG-positive prostate cancer would respond better to a MT-depolymerizing drug, such as a vinca alkaloid or Eribulin, both of which are FDA approved for other cancer indications, than to the MT, stabilizing taxanes, which are currently used as the standard of care. The role of ERG in decreasing taxane sensitivity is also supported by our results from ex vivo treatment of CTCs in which the presence of ERG (confirmed in CTCs and in the primary tumor) results in a lack of MT response to taxanes. Tiling mutant co-immunoprecipitation revealed that the PNT domain of ERG—initially identified in the Drosophila melanogaster protein pointed (Pnt), and conserved among multiple ETS-domain proteins [59] — mediates tubulin binding. The PNT domain is important for ETS-domain protein homo-oligomerization [60] and heterodimerization [61] . Interestingly, we showed that removal of the PNT domain (ERG-ΔP) restores taxane sensitivity, suggesting that the physical association between ERG and tubulin is required for the resistant phenotype. The ETS domain is important for protein–DNA interactions required for transcriptional regulation. For ERG, both the PNT and the ETS domains are essential for homo- and heterodimeric complex formation [33] . In addition, in TMPRSS2 ERG-positive prostate cancer cells the ETS domain is essential for the interactions between ERG and DNA repair proteins (for example, DNA-PKcs, Ku70, Ku80 and PARP1 (ref. 10 )) or AR [51] . Our data showed that, although the ETS domain was not essential for the ERG–tubulin interaction, its removal resulted in enhanced taxane sensitivity suggesting that ERG dimerization or a domain-specific transcriptional mechanism contributes to the overall ERG-mediated taxane resistance. Finally, the association between ERG and taxane resistance may also lead to enhanced androgen signalling in the context of taxane chemotherapy. We and others have shown that taxanes inhibit AR trafficking to the nucleus and AR signalling [36] , [61] , [62] , downstream of drug-induced MT stabilization. Interestingly, we have also shown that ERG cooperates with AR to regulate genes important for cell invasion and dedifferentiation in prostate cancer [14] . Herein, we show that ERG expression affects the ability of taxanes to target MTs, suggesting that AR inhibition that occurs downstream of MT stabilization should be impaired in the presence of ERG. These data suggest that ERG acts upstream of AR inhibition, further contributing to the taxane resistant phenotype. ERG rearrangement status was initially associated with response to the androgen biosynthesis inhibitor abiraterone acetate in a phase II clinical trial [41] , but this association was not confirmed in another study [63] . Future studies characterizing AR localization and function in the context of taxane treatment and ERG expression are required to resolve the interplay between ERG, MTs and AR, each of which representing an important target for prostate cancer treatment and all three together a novel actionable axis. In summary, our work identifies a new biological role for ERG, the product of the most common ETS gene rearrangement in prostate cancer, in taxane resistance. The identification of ERG as a biomarker predictive of response to MT inhibitors provides clinical rationale for treatment decisions and for patient selection for appropriate therapies, a step towards improving patient survival. Prospective clinical studies testing the concepts provided herein are warranted to transform these biological findings into clinical gains. Drug Treatment in vitro and in vivo Cabazitaxel was obtained from Sanofi in powder form. Prostate cell lines for this study were obtained from the American Type Culture Collection (Manassas, VA). RWPE (20 × 10 3 per well), DU145 (5 × 10 3 per well) and VCaP (20 × 10 3 per well) cells were seeded on 96-well tissue culture plates. To generate stable ERG overexpressing DU145 cells, the truncated ERG open reading frame was subcloned into a retroviral virus expression vector (pBABE; a kind gift from Dr William Hahn from the Broad Institute and the Dana Farber Cancer Center), which is equipped with an IRES-driving green fluorescent protein (GFP) expression [14] . Cell lines were treated with vehicle (0.5% ethanol) or escalating doses of cabazitaxel or docetaxel viability were assessed for cell viability (Cell Titer-Glo luminescent assay (Promega Corporation, Madison, WI) following the manufacturer’s protocol by incubating cells in a 96-well format in 1:1 v/v media to luminescent reagent for 10 min or apoptosis (caspase 3/7 activity (Caspase-Glo 3/7 Assay kit from Promega (Madison, WI) according to the manufacturer’s instructions. Cell viability dose response data were first normalized to data using the vehicle-treated control and then analysed using nonlinear regression in which the log (inhibitor) versus normalized response curves were generated and the IC 50 doses were calculated (GraphPad Software, San Diego California USA, www.graphpad.com ). Statistical significance of apoptosis data was determined using T-tests (Holm-Sidak method) provided by GraphPad Software. Xenografts were prepared by injecting 1 million DU145-ERG or DU145-GFP cells subcutaneously into 5-week male NU/J mice (Jackson Laboratories, Bar Harbor, Maine), and tumour volume was measured over an 8-week period (Weill Cornell Medical College Institutional Animal Care and Use Committee-approved protocol (#2008-0019). Two different studies were then performed using different clonal populations of DU145-ERG cells or DU145-GFP each. Tumours were allowed to grow to an average tumour volume of 150 mm 3 . For each study five mice bearing tumours from each cell type were randomized to treatment with cabazitaxel intraperitoneal dosing of 12 mg kg −1 or vehicle (5%ethanol/%PS80/glucose) every 6 days for 4 weeks. Body weight, tumour volume and cell viability based on caliper measurements (0.5236 × length × width) and bioluminescent imaging, respectively, were performed every 4 days to evaluate primary tumour growth. Cells were engineered to express luciferase using a transposable element vector (kind gift from John Ohlfest, University of Minnesota Medical School, Minneapolis, MN) as described previously [64] . On the day of imaging, we injected (intraperitoneal) 100 μl of D-Luciferin (75 mg kg −1 ) into anaesthetized mice. Ten minutes later the mice were placed on their ventral side and bioluminescence images were acquired with the IVIS Imaging System (Xenogen). Analysis was performed using LivingImage software (Xenogen). Images were acquired and analysed using LivingImage software (Xenogen) by measurement of the average photon flux (measured in photons s −1 cm −2 steradian −1 ) within a region of interest [18] . Mice were killed on week 10 (5 weeks after the first treatment and 1 week after the final treatment) and resected tumours were weighed, bisected and either immediately frozen in liquid nitrogen or prepared for formalin fixation and paraffin embedding (FFPE). Immunohistochemistry FFPE tissue sections were de-paraffinized and endogenous peroxidase was inactivated. Antigen retrieval was accomplished by heat/pressure cook using the Bond Epitope Retrieval Solution 1 (ER1) at 99–100 °C for 30 min (Leica Microsystems). Following retrieval, the sections were incubated sequentially with the primary antibody for 25 min, post-primary for 15 min and polymer for 25 min ending with colorimetric development with diaminobenzidine (DAB) for 10 min (Bond Polymer Refine Detection; Leica Microsystems). Antibodies used were ERG (1:100 Epitomics #28051), and ERG status was assessed as previously described [32] . In brief, subjective evaluation of ERG protein expression determined for each tumour core using a four-tier grading system: negative (0), weakly positive (1+), moderately positive (2+) and strongly positive (3+) in target cells above background (see Supplementary Table ). Fluorescent in situ hybridization ERG rearrangement was assessed using dual-color break-apart interphase FISH assay as described previously [11] , [65] , which involves labelling two probes that span the telomeric and centromeric neighbouring regions of the ERG locus. A nucleus that lacks ERG rearrangement demonstrates two pairs of juxtaposed red and green signals (which can form yellow signals). A nucleus with ERG rearrangement shows either split of one red-green (yellow) signal pair (indicating rearrangement through insertion) or one single red signal for the rearranged allele (indicating rearrangement through deletion). Transfection siRNA transfection was performed using Lipofectamine 2000 (Invitrogen, Carlsbad, CA) following the manufacturer’s recommended protocol. For the knockdown experiments, we used siERG (siGENOME Human ERG (2078)) or 100 nM control nonsilencing siGENOME siRNA (Thermo Scientific, Waltham, MA). For CLU mRNA knockdown, we used siCLU targeting the initiation site in exon II of human clusterin (5′-GCAGCAGAGUCUUCAUCAU-3′) and siSCR (5′-CAGCGCUGACAACAGUUUCAU-3′) for a control as previously described [66] . Following the indicated time, RNA was extracted and quantitative RT-PCR was performed. All experiments were performed in triplicate. Stable DU145 cells expressing ERG are described above and as previously described [17] . We generated inducible (tetracycline (Tet)-on) stable cell lines DU145 cells in which the level and timing of ERG expression is tightly controlled [67] using the pHERMES vector (kind gift of Dr William Hahn, The Broad Institute, Cambridge, MA) that were adapted with truncated ERG described in reference 14 (ref. 14 ) and that contain a non-leaky tetracycline response element-minimal CMV promoter together with the CMV-driven tetracycline controlled transactivator TetOn gene. The retroviral construct was transfected into 293FT cells with Lipofectamine 2000 according to the manufacturer’s instructions. The virus was harvested 72 h later and used to infect DU145 cells. GFP-positive cells (ERG over-expressing or empty vector) were enriched using GFP-based cell sorting using a FACS Aria-II Sorter. The different Flag-tagged ERG protein constructs have been previously described [10] and were a kind gift of Dr J. Chad Brenner (University of Michigan). Immunoblot analysis Protein lysates were prepared in the RIPA buffer (radioimmunoprecipitation assay lysis buffer) supplemented with protease inhibitor cocktail and phosphatase inhibitors (Thermo Scientific, Waltham, MA). The total protein concentration of the soluble extract was determined using the BCA protein assay Kit (Thermo Scientific). Each protein sample (30μg) was resolved to SDS–polyacrylamide gel electrophoresis (SDS–PAGE), transferred onto a polyvinylidene difluoride membrane (Millipore) and incubated overnight at 4 °C with primary antibodies. The antibodies used were ERG (1:2,000 Abcam, #ab133264); JUN (1:1,000 Santa Cruz, sc-1694X); rabbit anti-FLAG (1:1,000 Sigma, F7425); pan-cytokeratin (1:1,000 BioLegend, clone C-11 cat # 628602 and Lot # B181240); αtubulin (1:1,000 Sigma, #T6199) and GAPDH (1:10,000 Abcam, sb-75834). Following three washes with TBS-T, the blot was incubated with a horseradish peroxidase-conjugated secondary antibody and immune complexes were visualized by enhanced chemiluminescence detection (ECL plus kit, GE Healthcare, UK). The blot was reprobed with a monoclonal antibody against beta-actin (1:10,000 Sigma). Total protein was extracted and separated by gel electrophoresis. Protein was then transferred to nitrocellulose membranes and probed overnight using the appropriate primary antibodies. Tubulin polymerization assay Tubulin polymerization assay was performed as described before [20] . In brief, cells were plated in 24-well plates and then treated with different concentrations of either docetaxel or cabazitaxel overnight; after the treatment, cells were washed with warm phosphate buffered saline and lysed at 37 °C for 10 min with 100 μl of hypotonic buffer (1 mM MgCl 2, 2 mM EGTA, 0.5% Nonidet P-40) supplemented with 7 × protease inhibitor cocktail (Roche Diagnostics). The lysates were transferred to an Eppendorf tube and spun down at 14,000 r.p.m. for 10 min at room temperature; the supernatants containing soluble tubulin (cytosolic) were transferred to another tube, separating them from the pellets containing polymerized tubulin (cytoskeletal). The cytosolic and cytoskeletal components were resuspended into SDS sample buffer and boiled for 5 min. Twenty microlitres of each sample was separated via electrophoresis, and proteins were transferred onto polyvinylidene difluoride membranes; anti α-tubulin antibody (Sigma) was used as a primary antibody and an antibody compatible with the Odyssey Imaging System from LICOR Biosciences (Lincoln, NE) was used as a secondary antibody. Densitometry was performed with Image J software (National Institute of Health, Bethesda, MD, USA). Immunofluorescence Cells were plated on 1.5 mm coverslips (Electron Microscopy Services, Hatfields, PA, USA); after the drug treatment, cells were fixed with Phemo buffer (68 mM PIPES, 25 mM HEPES, 15 mM EGTA, 3 mM MgCl 2 , 10% DMSO) supplemented with 3.7% formaldehyde, 0.05% glutaraldehyde and 0.5% Triton X-100 and subsequently blocked with 10% Normal Goat Serum (Jackson ImmunoResearch, PA, USA). An anti α-tubulin antibody (Sigma) was used as a primary antibody followed by an anti-mouse Alexa 568 secondary antibody; DAPI was used for nuclear counterstain. For fluorescently labelled paclitaxel, live cells were permeabilized with 0.5% triton X-100 for 60 s, followed by incubation with Flutax-2 (kind gift of Dr Diaz) for 5 min. Images were acquired using Yokogawa CSU-X1 spinning disk confocal microscope under a × 100 objective (Zeiss, Germany). Flow cytometry Live cells were collected and incubated with an anti-P-gp primary antibody (MRK16, Enzo Live Science) for 1 h at 4 °C, followed by 30 min incubation with an Alexa Fluor 488 anti mouse secondary antibody. Data were acquired with LSR II system (BD Biosciences, San Jose, CA, USA) and results were analysed with FlowJo flow cytometry analysis software (TreeStar, Ashland, OR, USA). Drug accumulation assay Cells were plated in a 24-well plate and treated with 100 nM C-14-labelled cabazitaxel; after the treatment, cells were washed with cold PBS and collected, and the cell suspension was then diluted 1/10 in scintillation cocktail (Ecoscint A, National Diagnostics). The amount of intracellular radio labelled drug was detected with Scintillation Counter (LS650 Multipurpose scintillation counter, Beckman Coulter) and measured as count per minute (CPM) and normalized over cell number (CPM/100,000 cells). Microtubule co-sedimentation assay In brief, 1 mg of total cell lysate was first precleared by high-speed centrifugation. The pellet (HSP) containing mostly insoluble cell debris was discarded after loading a small amount on the gel to identify whether there was a significant loss of androgen receptor in the cell debris, whereas the supernatant (HSS) was supplemented with exogenous purified bovine brain tubulin (Cytoskeleton) reconstituted at a final concentration of 10 μmol l −1 in the presence of 1 mmol l −1 GTP and 20 μmol l −1 paclitaxel (PTX) and subjected to a cycle of polymerization for 30 min at 37 °C. Samples were centrifuged at 100,000 × g for 30 min at room temperature, and the warm supernatant (WS) was separated from the warm pellet (WP), which was resuspended in an equal volume of PEM buffer. Equal volumes from each respective fraction were loaded onto a SDS-PAGE and transferred and immunoblotted with antibodies against ERG or tubulin. EB comet imaging assays Tetracycline-inducible ERG overexpressing DU145 cells were plated on 3 cm dishes and infected with GFP-EB1ΔC lentiviral particles. EB1ΔC (referred to throughout the manuscript as EB1 for simplicity) is an EB1 construct truncated at amino acid 248 that does not interact with other +TIP proteins [68] . This construct had a better signal-to-noise ratio than full-length EB1, as determined empirically. The cells were imaged 2 days post infection to measure the dynamicity of MT ends labelled with GFP-EB1ΔC. Cells were pretreated with vehicle (DMSO) or Docetaxel for 1 h at 37 °C before imaging. Images were acquired every 0.5 s for a total of 1 min for each time-lapse movie. Computational analysis of MT dynamics using EBs All image analysis was performed using ClusterTrack, an algorithm that has been described in detail previously [31] , [69] . In brief, this approach can track thousands of EB-EGFP comets that are visible in images within a time-lapse sequence. Imaging these comets allows the detection of spatial patterns of MT dynamics. The algorithm uses spatiotemporal clustering of EB-EGFP growth tracks to infer MT behaviours during phases of pausing and shortening. Parameters in ClusterTrack were as follows: s1=1.25, s2=3.5, k1=3.5, k2=1, search radius=6 pixels. Remaining conditions were set to defaults. Accuracy of comet tracking was verified by visual inspection of time-lapse movies. All parameters were calculated per cell. For each condition, 10 or more videos containing one or two cells are acquired. For statistical analysis, we used a permutation t -test (200 repetitions) to compare differences in the mean parameter values [69] . Metastatic castrate-resistant prostate cancer cohort The cohort consisted of 34 men with mCRPC, who were treated with docetaxel chemotherapy either at Royal Prince Alfred and Concord Hospitals ( n =28) or New York Presbyterian Hospital, Weill Cornell Medical College ( n =6). Patients were administered with docetaxel 75 mg m −2 3-weekly by the treating medical oncologist. They were seen every 3 weeks and had a serum PSA level performed. Consent was obtained for the collection of their archival formalin-fixed paraffin-embedded tissue from original diagnostic specimens. These tissues came from transrectal biopsies, trans-urethral resection of prostate, radical prostatectomy, bone biopsy and cell blocks from fine needle aspiration biopsy from metastases. The H&E slides were reviewed by a prostate cancer pathologist (J.K.) for evidence of representative cancer and were then stained according to standard protocols for ERG by immunohistochemistry [32] and/or TMPRSS2-ERG re-arrangement by FISH [32] . The ERG immunohistochemistry was scored by two observers one of whom was a pathologist. Both were blinded to clinical outcomes. Staining was predominantly nuclear with grade 1 intensity cytoplasmic expression seen in all positive cases. Cases were deemed positive if >50% of nuclei expressed ERG, however, of the eight ERG-positive cases, seven cases had 95% of nuclei positive for ERG and the remaining case was 60% nuclear positive. One case from a cytology cell block was positive for a TMPRSS2-ERG rearrangement, but negative on ERG immunohistochemistry most likely due to poor tissue quality. Response to docetaxel chemotherapy was measured by PSA criteria using PCWG2 criteria [70] . PCWG2 defines progressive disease as an increase of ≥25% (at least 2 ng ml −1 ) over the baseline value after 12 weeks of treatment, confirmed by a second PSA value at least 3 weeks later. Given that the PCWG2 criteria also suggest the assessment of PSA as a continuum, a waterfall plot was also used to illustrate the distribution of PSA changes over the course of docetaxel treatment against expression of TMPRSS2-ERG. All patients provided written informed consent, and the study was approved by human research ethics review committees at all participating institutions and was registered on the Australian New Zealand Clinical Trials Registry. Circulating tumour cells capture and ex vivo treatment assay Following written informed consent, peripheral blood from CRPC patients was collected in sodium citrate tubes (Greiner Bio-one, Monroe, NC, USA) and the Geometrically Enhanced Differential Immunocapture (GEDI) microfluidic device was used for CTCs isolation as previously described [43] , [71] . In brief, a total volume of 3 ml of peripheral blood was obtained from each of the patients evaluated; after chemical functionalization, each device was coated with a biotinylated anti PSMA antibody (clone J591, provided by Dr Neil Bander, Weill Cornell Medical College, NY, USA) and 1 ml of peripheral blood was processed through each of three separate GEDI devices. After CTC capture, the microfluidic devices were treated ex vivo with either Docetaxel 100 nM or Cabazitaxel 10 nM or DMSO as control for 24 h at 37 °C. After the treatment, the still viable CTCs were fixed with 2% formaldehyde in 50% Phem buffer (60 mM PIPES, 25 mM HEPES, 10 mM EGTA, 2 mM MgCl 2 ), permeabilized with 0.25% Triton X-100 (Sigma) and stained for our panel of markers: CD-45 (mouse anti CD-45 directly conjugated with Qdot 800, Invitrogen), ERG (rabbit anti ERG, Epitomics, followed by AlexaFluor 488 labelled goat anti rabbit secondary antibody), tyrosinated tubulin (rat tyr-tubulin, Millipore, followed by AlexaFluor 647 labelled goat anti rat secondary antibody) and cytokeratin (mouse anti pan-cytokeratin, Biolegend directly conjugated with CF594, Biotium); DAPI was used for DNA counterstain. High-resolution images were acquired using Yokogawa CSU-X1 confocal microscope with × 100 objective (Zeiss, Germany). CTCs were identified as DAPI+, CK+, CD-45− cells and all CTCs were evaluated for evidence of DTE, identified as MT bundling. Co-immunopreciptiation Cell lysates were prepared by lysing cells in buffer containing 50 mM Tris (pH 7.5), 120 mM NaCl, 0.5% NP-40, 5 mM EDTA and protease and phosphatase inhibitors (Thermo Scientific), as previously described [18] . Five hundred micrograms of total protein extract was incubated with 5 μg of anti-ERG (Abcam, #ab133264), DM1a (tubulin, Sigma, #T6199), Flag (Sigma #F7425) or control IgG (Epitomics, #ISO-5115) overnight and precipitated protein was analysed using western blot analyses for the indicated proteins. An aliquot of cell lysate before immunoprecipitation was used for the input sample. How to cite this article: Galletti, G. et al. ERG induces taxane resistance in castration-resistant prostate cancer. Nat. Commun. 5:5548 doi: 10.1038/ncomms6548 (2014).